Ultrafast observation of critical nematic fluctuations and giant magnetoelastic coupling in iron pnictides Many of the iron pnictides have strongly anisotropic normal-state characteristics, important for the exotic magnetic and superconducting behaviour these materials exhibit. Yet, the origin of the observed anisotropy is unclear. Electronically driven nematicity has been suggested, but distinguishing this as an independent degree of freedom from magnetic and structural orders is difficult, as these couple together to break the same tetragonal symmetry. Here we use time-resolved polarimetry to reveal critical nematic fluctuations in unstrained Ba(Fe 1− x Co x ) 2 As 2 . The femtosecond anisotropic response, which arises from the two-fold in-plane anisotropy of the complex refractive index, displays a characteristic two-step recovery absent in the isotropic response. The fast recovery appears only in the magnetically ordered state, whereas the slow one persists in the paramagnetic phase with a critical divergence approaching the structural transition temperature. The dynamics also reveal a gigantic magnetoelastic coupling that far exceeds electron–spin and electron–phonon couplings, opposite to conventional magnetic metals. In the electronic nematic state of the iron pnictides, the high-temperature tetragonal symmetry ( C 4 ) of the system is lowered to an orthorhombic one ( C 2 ) at the temperature T S through the divergence of nematic fluctuations ( Fig. 1a ). The associated nematic-order parameter φ has therefore Ising ( Z 2 ) character (two discrete values) [1] , [2] , [3] . Its coupling to other degrees of freedom, such as magnetic fluctuations, lattice orthorhombicity and orbital order [4] , thus gives rise to anisotropies in several quantities—electrical and thermal transport, orbital occupation, optical conductivity and magnetic susceptibility [5] , [6] , [7] , [8] , [9] , [10] , [11] , [12] , [13] . In most materials, the nematic transition usually takes place very close to a magnetic transition at T N ≤ T S , giving rise to a (0, π )/( π , 0) spin-striped state [14] . The challenge arises on how to underpin the anisotropy from electronic nematicity and disentangle it from various different, although cooperative, contributions [1] , [2] , [3] , [4] , [15] , [16] . 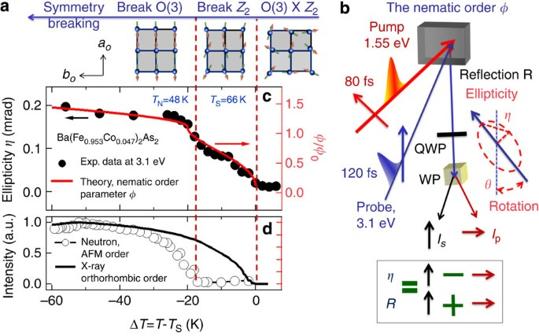Figure 1: A laser-based polarimetry technique measures the ellipticityη. It is directly proportional to the Ising-nematic-order parameter,φ, in Ba(Fe1−xCox)2As2systems. (a) Schematics of the establishment of the Ising-nematic phase via spontaneous tetragonal symmetry breaking, illustrated in theabplane. At high temperatures, there exists aO(3) spin-rotational symmetry along with the Ising-nematicZ2symmetry associated with the double degeneracy of the magnetic ground state, corresponding to magnetic stripes with either (0,π) or (π, 0) modulation. Below the tetragonal-to-orthorhombic transition temperatureTS, this emergentZ2symmetry is broken, but theO(3) symmetry is preserved untilT≤TN, when long-range magnetic order sets in. AtTS, the system also develops orbital and structural order. (b) As illustrated, the ellipticity of the reflected beam is detected by passing the reflected beam through a quarter-wave plate (QWP), with its axis oriented at 45° with respect to the verticalsaxis, and a polarization-dependent beam splitter (wollaston prism, WP) to spatially separate theS- andP-polarized components (see Methods section). The anisotropy componentηis measured fromIS−IPand the isotropic contributionRfromIS+IP. (c) The measured temperature-dependentη(black solid dots) and the calculated normalized nematic-order parameterφ/φ0for thex=0.047 sample agree very well. The coupling between the nematic- and magnetic-order parameters—black empty dots shown indextracted via neutron scattering—is manifested by the hump inφatTN=48 K. The coupling betweenφand the lattice gives rise to a non-zero orthorhombicity atTS=66 K, as found by X-ray scattering—black line ind. Figure 1: A laser-based polarimetry technique measures the ellipticity η . It is directly proportional to the Ising-nematic-order parameter, φ , in Ba(Fe 1− x Co x ) 2 As 2 systems. ( a ) Schematics of the establishment of the Ising-nematic phase via spontaneous tetragonal symmetry breaking, illustrated in the ab plane. At high temperatures, there exists a O (3) spin-rotational symmetry along with the Ising-nematic Z 2 symmetry associated with the double degeneracy of the magnetic ground state, corresponding to magnetic stripes with either (0, π ) or ( π , 0) modulation. Below the tetragonal-to-orthorhombic transition temperature T S , this emergent Z 2 symmetry is broken, but the O (3) symmetry is preserved until T ≤ T N , when long-range magnetic order sets in. At T S , the system also develops orbital and structural order. ( b ) As illustrated, the ellipticity of the reflected beam is detected by passing the reflected beam through a quarter-wave plate (QWP), with its axis oriented at 45° with respect to the vertical s axis, and a polarization-dependent beam splitter (wollaston prism, WP) to spatially separate the S - and P -polarized components (see Methods section). The anisotropy component η is measured from I S − I P and the isotropic contribution R from I S + I P . ( c ) The measured temperature-dependent η (black solid dots) and the calculated normalized nematic-order parameter φ / φ 0 for the x =0.047 sample agree very well. The coupling between the nematic- and magnetic-order parameters—black empty dots shown in d extracted via neutron scattering—is manifested by the hump in φ at T N =48 K. The coupling between φ and the lattice gives rise to a non-zero orthorhombicity at T S =66 K, as found by X-ray scattering—black line in d . Full size image Ultrafast dynamics of the nematic-order parameter φ in iron pnictides has not been measured thus far, despite the fact that this approach can potentially reveal dynamic and critical fluctuations associated with the establishment of the new phase. The time resolution also disentangles the various coupled order parameters based on their distinct relaxation dynamics subsequent to being suddenly driven out of equilibrium. Such a femtosecond (fs)-resolved approach can reveal information hidden inside the time-averaged signals obtained from static measurements. Prior ultrafast experiments in iron pnictides mostly concentrated on laser-induced melting of the superconducting and spin density wave (SDW) gaps and on charge-quasiparticle dynamics, but provided little insight into nematicity, as it is not known how to resolve the φ -order-parameter dynamics [17] , [18] , [19] , [20] , [21] , [22] . Recently, linear polarization spectroscopy from the far-infrared up to 2 eV revealed an anisotropy of the static conductivity along the a and b orthorhombic directions ( Fig. 1a ), along (0, π ) and ( π ,0) directions, thus paving a way to optically probe the Z 2 Ising order parameter [9] , [10] . However, two key issues remain before one can access the unexplored ultrafast regime: first, probing the anisotropy in the ultraviolet region is most critical, as this minimizes the contamination of ultrafast polarization signals by spurious effects, for example, spectral weight transfer associated with pump-induced Fermi-surface reconstruction and transient filling of the mid-infrared SDW gaps (see Methods section). Thus far, optical anisotropy above 2 eV could not be observed with conventional broadband polarization optics [9] . Second, to access the ‘spontaneous’ order φ , it is critical to study unstrained single crystals. Even a small external strain will smear out the well-defined critical temperature, predicted at T S , because of the large nematic susceptibility [5] , [6] . This article characterizes ultrafast relaxation of the Ising-nematic-order parameter φ following non-equilibrium photoexcitation at 1.55 eV of unstrained Ba(Fe 1– x Co x ) 2 As 2 , by using laser-based, fs-resolved polarimetry probe centred at the near-ultraviolet region, at 3.1 eV (see Methods section). A two-step polarization recovery with fast ( τ fast ) and slow ( τ slow ) relaxation times is observed only in the anisotropic response Δη. Such two-step relaxation dynamics is absent in the measured response Δ R / R that mostly arises from the isotropic transient electron and lattice relaxations. In both parent ( x =0.00, with T S ≈ T N =136 K) and underdoped ( x =0.047, with T S =66 K and T N =48 K) single crystals (see Methods section) [23] , we are able to separate the contributions to the anisotropy relaxation: the long-range magnetic order, τ fast , is present only below T N , whereas the nematic fluctuations, τ slow , persist even in the paramagnetic orthorhombic phase. In the parent compound, a sharp increase of τ slow is clearly observed on approaching T S , which is indicative of critical divergence of nematic fluctuations. τ slow is also observed to increase close to T S in the underdoped compound, despite the smaller signal-to-noise ratio. A quasi-equilibrium, three-temperature (3T) model reproduces the first few picosecond dynamics and reveals, particularly, a gigantic magneto-elastic coupling that far exceeds both e -spin and e -phonon couplings, opposite to what is observed in magnetic metals [24] . Our direct measurement of time-dependent anisotropy thus establishes the presence of an independent electronic nematic degree of freedom in iron pnictides, and bridges the gap between quantum nematic matter and technologically interesting functionalities. The demonstrated ultrafast polarimetry approach provides a versatile and powerful spectroscopic tool to investigate the electronic nematicity and disentangle its coupling with other order parameters. Laser-based static polarimetry of nematic-order parameter φ As illustrated in Fig. 1b , when a linearly polarized optical field, oriented at 45° with respect to the orthogonal axes of different complex refractive indices and , is incident on the sample surface, an elliptically polarized light ( η ) with a rotated polarization plane ( θ ) is reflected (see Methods section). A complex angle =θ+ i η can be obtained by expanding the solution of the Fresnel equation with respect to α =Δ (defined as ( <<1): and is directly proportional to Δ , that is, ∝ φ. As the real and imaginary parts of are connected via Kramers–Kronig relations, we focus on the imaginary part of , η , to extract information about φ . We obtain η by subtracting the S- and P -polarized components ( I S − I P )/2( I S + I P ), after dividing by the surface reflection R = I S + I P , a measure of the isotropic response (black box). The result for unstrained, underdoped Ba(Fe 0.953 Co 0.047 ) 2 As 2 (black dots) is shown in Fig. 1c . Decreasing the temperature, η shows a gradual increase only below T S =66 K and exhibits a distinct increase across ≈ T N =48 K. This temperature dependence reveals a coupling between the nematic-order parameter φ and the magnetic- and orthorhombic-order parameters measured with X-ray and neutron scattering ( Fig. 1d ) [25] . Furthermore, a quantitative comparison of the measured temperature profile of η ( T ) with the theoretically predicted behaviour of φ ( T ) shows a good agreement. In this calculation, the degeneracy of the magnetic ground state, allied to magnetic fluctuations, gives rise to a non-zero nematic-order parameter at T S , which is enhanced at T N due to the feedback effect on the magnetic spectrum (see Fig. 1a and Methods). The anisotropic optical conductivity observed at such high energies, ~3 eV, arises most likely from the non-equivalent occupations of the d xz and d yz Fe orbitals, which is proportional to the nematic order induced by magnetic fluctuations. It is noteworthy that the full temperature dependence of φ measured here has been inaccessible with various other probes, for example, due to the inapplicability of magnetometry in the SDW phase [13] and due to the limited signal-to-noise ratio in polarized photoemission [8] . Ultrafast spectroscopy measurements We start with the parent (undoped) compound. The fs-resolved ellipticity change Δ η is shown on a logarithmic scale as a function of time delay in Fig. 2a at 4 K under pump fluence of 115 μJ cm −2 . Ultrafast photoexcitation results in the sudden softening of the nematic order, revealed by a negative change Δ η <0, which is followed by a bi-exponential recovery composed of an initial fast relaxation of τ fast ~1.2 ps and a subsequent slow one of τ slow ~28 ps. The most salient feature in Fig. 2 is the striking difference in temporal profiles between the polarization Δ η and the simultaneously probed reflectivity Δ R / R . This difference persists both in the fs and in the subsequent extended 100 ps time intervals. The inset of Fig. 2a focuses on the first 1.2 ps and reveals a delayed rise Δ τ rise of Δ η (black dots) as compared with Δ R / R (red shade). This delay indicates a fast electron thermalization ~150 fs before the softening of the nematic order. Three key properties of the relaxation times τ fast and τ slow of Δ η are seen following this initial thermalization: (i) both relaxations are absent in the Δ R / R decay profiles dominated by cooling of hot electrons and lattice, as Δ R / R originates from thermally induced band structure renormalization. The clear difference in the time evolution of η strongly points to a separate physical origin of the measured anisotropy. (ii) The τ fast and τ slow components exhibit a distinctly different dependence on temperature ( Fig. 2b,c ): τ fast displays little variation between 4 and 130 K, whereas τ slow shows a much faster relaxation at low temperatures ( T =4 K ) than at temperatures ( T =130 K) slightly below T S =136 K. This trend is clearly visible by following the τ slow dynamics (blue shades) at various temperatures, shown in Fig. 2d . A detailed fitting of the temperature dependence of the two-step recovery (red lines, also see Supplementary Note 3 and Supplementary Fig. 1 ) reveals that τ slow is mostly constant up to near T S , where it sharply increases in a way that indicates critical divergence near the phase transition (inset). As the structural transition is second order while the magnetic one is first order in the parent compound, the critical slowing down behaviour in Fig. 2d must come only from the structural transition. In contrast, Δ R / R mostly exhibits a temperature-independent decay profile: the 4K and 130K traces (red shade, Fig. 2b,c ) are almost identical. This distinct behaviour of the anisotropic-only response rules out effects such as gap opening in the density of states and phonon fluctuations as the origin of observed critical slowing down in τ slow . We attribute this remarkable anisotropic response to the predicted divergence of nematic correlation at T S (refs 4 , 11 ). (iii) The photoinduced Δ η amplitude quickly diminishes above T S , but not Δ R / R , which again corroborates the nematic origin of the observed transient η signal. It is noteworthy that unlike Δ η , Δ R / R also shows a periodic oscillation of ~120 fs, which arise from the As–As optical phonon [18] . 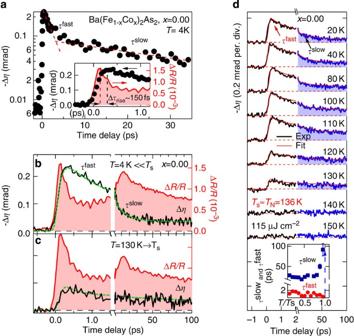Figure 2: Ultrafast photoinduced dynamics of the nematic-order parameter in the parent compound BaFe2As2. (a) Ultrafast photoinduced change in the ellipticity ΔηatT=4 K for 35 ps and for the first 1.2 ps of time delay (black dots, inset). Δηexhibits a double-exponential time-dependent recovery with time constantsτfast=1.2 ps andτslow=28 ps (red dashed lines). The inset reveals a delayed rise Δτriseof Δη(black dots) compared with ΔR/R(red shade), which indicates a faster electron thermalization ~150 fs before the softening of the nematic order. (b,c) The photoinduced ellipticity Δη(back lines) and ΔR/R(red shades) for the first 1.5 ps and for the extended time scales of 100 ps (split axis) at two temperatures 4 K (b) and 130 K (c). Green dash lines: data fittings (seeSupplementary Note 3). (d) Detailed temperature dependence of the photoinduced ellipticity Δηfor the first 2 ps (black lines) and extended 100 ps (blue shades, split axis), shown together with double-exponential fittings (red lines). Pump fluence used for all traces is 115 μJ cm−2. The extractedτfast(red circles) andτslow(blue squares) with error bars, defined as the s.d. in the fitting, are presented in the inset as a function of the normalized temperatureT/TS. Note the critical slowing down in theτslowrelaxation time atTS(blue dashed line). Figure 2: Ultrafast photoinduced dynamics of the nematic-order parameter in the parent compound BaFe 2 As 2 . ( a ) Ultrafast photoinduced change in the ellipticity Δ η at T =4 K for 35 ps and for the first 1.2 ps of time delay (black dots, inset). Δ η exhibits a double-exponential time-dependent recovery with time constants τ fast =1.2 ps and τ slow =28 ps (red dashed lines). The inset reveals a delayed rise Δ τ rise of Δ η (black dots) compared with Δ R / R (red shade), which indicates a faster electron thermalization ~150 fs before the softening of the nematic order. ( b , c ) The photoinduced ellipticity Δ η (back lines) and Δ R / R (red shades) for the first 1.5 ps and for the extended time scales of 100 ps (split axis) at two temperatures 4 K ( b ) and 130 K ( c ). Green dash lines: data fittings (see Supplementary Note 3 ). ( d ) Detailed temperature dependence of the photoinduced ellipticity Δ η for the first 2 ps (black lines) and extended 100 ps (blue shades, split axis), shown together with double-exponential fittings (red lines). Pump fluence used for all traces is 115 μJ cm −2 . The extracted τ fast (red circles) and τ slow (blue squares) with error bars, defined as the s.d. in the fitting, are presented in the inset as a function of the normalized temperature T / T S . Note the critical slowing down in the τ slow relaxation time at T S (blue dashed line). 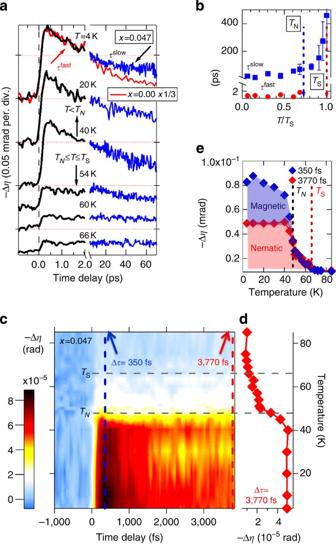Figure 3: Ultrafast photoinduced dynamics of the nematic-order parameter in (underdoped) Ba(Fe0.953Co0.047)2As2. (a) Detailed temperature dependence of the ultrafast photoinduced ellipticity change Δηforx=0.047 samples for the first 2 ps (black lines) and for extended time scales of 100 ps (blue lines, split axis), shown together with the 4 K ellipticity trace forx=0 sample (red lines). The pump fluence used for all six traces is 115 μJ cm−2. (b) The extractedτfast(red circles) andτslow(blue squares) with error bars, defined as the s.d. in the fitting, are presented as a function of the normalized temperatureT/TS. Note the critical slowing down in theτslowrelaxation time atTS(red dashed line). (c) A false colour image of the time-resolved ellipticity change Δηfor thex=0.047 sample as function of temperature, showing distinct transitions at bothTNandTS. (d) Temperature dependence of the photoinduced Δηat Δτ=3,770 fs. (e) Temperature dependence of the photoinduced Δηat two time intervals Δτ=350 fs (blue solid diamonds) and 3,770 fs (red solid diamonds), following photoexcitation. The blue and red shaded regions show the inferred contributions to the nematicity coming from the magnetic-order parameters (marked as magnetic) and other Ising-nematic contributions (marked as nematic), respectively. Full size image Figure 3a presents ultrafast Δ η measurements on the x =0.047 sample, which undergoes separate magnetic and structural transitions ( T N =48 K and T S =66 K, respectively). At 4 K and pump fluence of 115 μJ cm −2 , we again observe a bi-exponential relaxation behaviour similar to the x =0.00 sample. However, at T =54 K slightly above T N =48 K, the τ fast component disappears, while the τ slow relaxation persists. In addition, the photoinduced ultrafast ellipticity dynamics at T =60 K and T =66 K that approach the structural transition temperature (red line) exhibits a slower τ slow relaxation time as compared with 4, 10, 40 and 54 K. A detailed fitting of the temperature dependence of the two-step recovery ( Fig. 3b ) again shows a slowing down of τ slow near T S , observed despite our smaller signal-to-noise ratio as compared with the parent compound. The detailed temperature dependence of Δ η shown in Fig. 3c confirms that the τ fast component exclusively appears below T N and, therefore, originates from the long-range magnetic-order contribution to the anisotropy. In Fig. 3d , the τ slow component (white area in Fig. 3c , shown at the fixed time delay Δ τ =3,770 fs), exhibits no change at low temperatures, begins to drop at ~ T N and then fades out only at T S =66 K. We therefore again attribute τ slow to the electronic nematicity, as there is no long-range magnetic order for T N < T < T S . Figure 3: Ultrafast photoinduced dynamics of the nematic-order parameter in (underdoped) Ba(Fe 0.953 Co 0.047 ) 2 As 2 . ( a ) Detailed temperature dependence of the ultrafast photoinduced ellipticity change Δ η for x =0.047 samples for the first 2 ps (black lines) and for extended time scales of 100 ps (blue lines, split axis), shown together with the 4 K ellipticity trace for x =0 sample (red lines). The pump fluence used for all six traces is 115 μJ cm −2 . ( b ) The extracted τ fast (red circles) and τ slow (blue squares) with error bars, defined as the s.d. in the fitting, are presented as a function of the normalized temperature T / T S . Note the critical slowing down in the τ slow relaxation time at T S (red dashed line). ( c ) A false colour image of the time-resolved ellipticity change Δ η for the x =0.047 sample as function of temperature, showing distinct transitions at both T N and T S . ( d ) Temperature dependence of the photoinduced Δ η at Δ τ =3,770 fs. ( e ) Temperature dependence of the photoinduced Δ η at two time intervals Δ τ =350 fs (blue solid diamonds) and 3,770 fs (red solid diamonds), following photoexcitation. The blue and red shaded regions show the inferred contributions to the nematicity coming from the magnetic-order parameters (marked as magnetic) and other Ising-nematic contributions (marked as nematic), respectively. Full size image Figure 3e compares the photoinduced Δ η dynamics in the x =0.047 sample versus temperature at two fixed time delays Δ τ =350 and 3,770 fs. Although these two Δ η amplitudes are different below T N , they coincide above T N , and both then diminish at T S . This salient feature allows us to estimate the ratio between the contributions to the nematicity from the magnetic order versus other Ising-nematic contributions. The difference of the two amplitudes Δ η | Δ τ =350 fs −Δ η | Δ τ =3,770 fs measures the pure magnetic-order contribution, which sets in only below T N (blue shaded region). The contribution to the anisotropy from the nematic-order parameter is characterized by Δ η | Δτ =3,770 fs (red shaded region), which begins to increase at T S , exhibits a kink at T N due to the magnetic feedback effect and shows little variation deep inside the SDW phase. The comparable magnitude between the two above contributions indicates a substantial spin influence on the nematicity, which we address next. Comparing fs-resolved nematicity and charge-carrier dynamics Analysing the fs-resolved nematicity and charge-carrier dynamics in terms of a transient temperature description reveals key information about the coupling between the different reservoirs. The transient temperature T e associated with the electron heat bath after ultrafast photoexcitation is proportional to the differential reflectivity profile, Δ T e ∝ Δ R / R (Δ τ ) as established in many prior ultrafast studies of metals [24] , [26] , after subtracting a local maximum at ~10 ps here. Below T N , we introduce a reservoir temperature T m characterizing the magnetic–nematic phase. In this regime, both the nematic- and the magnetic-order parameters contribute to the anisotropy, whereas the latter dominates the time evolution during the first few ps. From the temperature dependence of the static η ( Fig. 1c ) and the photoinduced changes Δ η , we extract the temporal profile of T m from the ultrafast data ( Supplementary Note 4 and Supplementary Fig. 2 ). 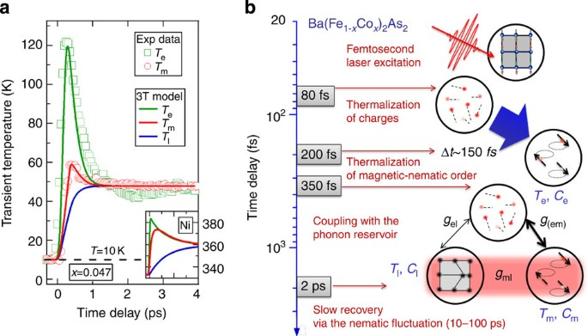Figure 4: Ultrafast photoinduced transient cooperative processes in iron pnictides. (a) The measured and calculated ultrafast transient temperature changes up to 4 ps for the electron (Te), lattice (Tl) and magnetic–nematic (Tm) heat baths atTi=10 K. Shown together in the inset is the result from elemental nickel for comparison (T=300 K,TC=631 K). (b) A unified picture emerges for transient photo-driven cooperative processes in iron-pnictide systems with the respective time scales extracted from our analysis. The illustration refers to low temperaturesT<TN,TSunder the 80 fs photoexcitation. It depicts, in this order: the electron thermalization and cooling, the magnetic–nematic-order thermalization, the lattice heating through strong spin–optical phonon coupling, the slow recovery of the nematic order via its own fluctuation diverging atTSand the final relaxation back toT=10 K by heat diffusion. Figure 4a shows T e ( t ) (green squares) and T m ( t ) (red circles) for the first 4 ps in the x =0.047 sample at an initial temperature 10 K and pump fluence of 172 μJ cm −2 . T e ( t ) rises first during the 80 fs ultrafast photoexcitation via laser heating of the electronic subsystem, followed by an increase of the magnetic–nematic reservoir temperature T m via heat transfer from the electron reservoir. The most salient feature is that T m decays far before equilibrating with T e —that is, before reaching T e ( t ). This is opposite to what is observed in ferromagnetic metals such as nickel [24] , [26] , where (inset Fig. ) the magnetic and electron subsystems first reach the same temperature and then lock together to decay towards an isothermal regime of the same heat-bath temperature with phonons ( T l ), that is, T m does not decrease before equilibrating with electrons ( Supplementary Note 5 ) [24] , [26] . This behaviour in conventional metals is due largely to the weak spin–phonon interaction compared with e -phonon and e -spin couplings, that is, g ml << g el , g em . The observation of an opposite trend in iron pnictides underpins an unusually strong spin–phonon coupling, that is, g ml ≫ g el , g em . This result follows naturally from a magnetic–nematic state, where the nematic-order parameter mediates the coupling between spin and lattice degrees of freedom, and is seen by the direct comparison of experimental data in the two material systems without any modelling ( Supplementary Discussion ). We also performed controlled measurements at a substantially lower pump fluence, which indicate that sample heating effects are not the dominant mechanism ( Supplementary Fig. 3 ). Figure 4: Ultrafast photoinduced transient cooperative processes in iron pnictides. ( a ) The measured and calculated ultrafast transient temperature changes up to 4 ps for the electron ( T e ), lattice ( T l ) and magnetic–nematic ( T m ) heat baths at T i =10 K. Shown together in the inset is the result from elemental nickel for comparison ( T =300 K, T C =631 K). ( b ) A unified picture emerges for transient photo-driven cooperative processes in iron-pnictide systems with the respective time scales extracted from our analysis. The illustration refers to low temperatures T < T N , T S under the 80 fs photoexcitation. It depicts, in this order: the electron thermalization and cooling, the magnetic–nematic-order thermalization, the lattice heating through strong spin–optical phonon coupling, the slow recovery of the nematic order via its own fluctuation diverging at T S and the final relaxation back to T =10 K by heat diffusion. Full size image Modelling of the first few ps ultrafast dynamics For further understanding, we simulate the obtained ultrafast dynamics using a 3T model via a set of coupled differential equations describing energy flow between three reservoirs, which describes transient couplings among the electron ( T e ), lattice ( T l ) and spin–nematic ( T m ) heat baths with corresponding coupling constants g ij following pumping with a rate P ( t ) of 673 J mol −1 by the 80 fs Gaussian laser pulses over the excited volume (see Methods section). This model is an extension of the two-temperature model that describes the ( T e ) and ( T l ) thermal relaxation in metals by adding T m . The best-fit coupling constants are g em =3.16 × 10 17 W m −3 ˙K, g ml =13.3 × 10 17 W m −3 ˙K and g el =0.033 × 10 1 W m −3 ˙K. The results of this calculation, shown in Fig. 4a , agree very well with the experiment, and reveal, particularly, a giant ratio g ml / g em larger than that in nickel by ~100 times for the best-fit values and by a lower bound of ~64 times considering error bars (Methods). A unified picture emerges for transient photo-driven cooperative processes in iron pnictides, illustrated in Fig. 4b for low temperatures T < T S , T N : ultrafast photoexcitations during 80 fs, shorter than the As–As optical phonon period, suddenly and strongly alter the thermodynamic equilibrium between various reservoirs. (i) During or immediately following the pulse, electron–electron collisions lead to decoherence and the quick establishment of a quasi-thermal distribution of charge carriers after an electron thermalization time ~200 fs. (ii) Next, the electrons cool down through energy transfer to the other reservoirs. Spin–electron interaction gives rise to the softening of the spin–nematic order, which leads to the delayed negative rise Δ τ rise ~150 fs of the thermalized magnetic–nematic order. (iii) The subsequent fast decay, up to ~2 ps of T m , indicates lattice heating through strong spin–optical phonon coupling, which reaches an isothermal regime of lattice, electron, magnetic–nematic reservoirs, still higher than the equilibrium lattice temperature before the pump. (iv) The slow recovery of the nematic order proceeds within ~20–100 ps via the nematic fluctuation channel, and the system finally relaxes back to the equilibrium lattice temperature by heat diffusion between the laser pulses (1 ms). The above reservoir temperature analysis is limited when describing the nematic fluctuations on time intervals of tens of ps, as clearly shown by the raw data presented in Figs 2d and 3a . This is the reason why here our modelling mainly focuses on the fast, few-ps components, where the magnetic softening and relaxation are the main nonlinear mechanisms, and, thereby, provides insights into the previously inaccessible couplings among various reservoirs. Our results should motivate the development of a microscopic theory for non-equilibrium quantum dynamics and critical phenomena of the electronic nematicity, a very challenging problem at the moment. In addition, we should note that a comparison of the ultrafast dynamics in iron pnictides to specifically chosen antiferromagnetic metals with similar transition temperatures and large electron–spin coupling g em exceeding g el and g ml would be desirable. However, this is a rare combination and we are not aware of such a material to compare our results. On the other hand, ferromagnetic metals such as nickel have long been established as a prominent example with g em exceeding g el and g ml . Our results reveal some important issues that warrant further investigations: the microscopic origin of the transient anisotropic response and its pronounced differences from the isotropic signals; the universality of the demonstrated ultrafast approach based on time-resolved critical dynamics to study other quantum nematic matter with various dopings/compositions [27] . The electronic nematicity can be further explored via complementary techniques to be sensitive to anisotropic SDW gaps, such as ultrafast near- and mid-infrared spectroscopy [28] , [29] , [30] , [31] . Iron pnictides may provide another playground for exploring quantum fs tuning of exotic ground states in complex materials [32] , [33] , [34] . Ba(Fe 1- x Co x ) 2 As 2 growth and characterization Single crystals of Ba(Fe 1– x Co x ) 2 As 2 , x =0.00 and 0.047, were grown out of a (Fe 1– y Co y )As flux, using conventional high-temperature solution growth techniques [23] , [35] . For the x =0.00 parent compound, small Ba chunks and FeAs powder were mixed together with 1:4 ratio. For the Co-substituted compound, small Ba chunks, FeAs powder and CoAs powder were mixed together according to the ratio Ba:FeAs:CoAs=1:3.75:0.25. Elemental analysis of the samples was performed using wavelength dispersive X-ray spectroscopy in the electron probe microanalyser of a JEOL JXA-8200 electron microprobe to determine the real Co concentration [35] . The x =0.047 sample undergoes a separate SDW transition at T N =48 K and a structural transition from tetragonal to orthorhombic phase at T S =66 K. For the x =0.00 sample, the T N and T S are almost indistinguishable in these measurements ~136 K (refs 25 , 35 ). Laser-based static polarimetry measurements Here we develop a more sensitive laser probe from a Ti:Sapphire oscillator (1.55 eV centre wavelength, ~100 fs pulse duration and 80 MHz repetition rate), that is, frequency—doubled to 400 nm (3.1 eV), as shown in Fig. 1b . In the definition above and in the Jones Matrix notation, the incident E-field ( s -polarized) and complex reflection E-field from the sample are E in =( E S , E P )=(1, 0) and E R =(1, ), respectively. The detection of the ellipticity η is achieved by passing the reflected beam through a quarter-wave plate, with its axis oriented at 45° with respect to the vertical s axis, and through a polarization-dependent beam splitter to spatially separate the S- and P-polarized components. The anisotropy η is calculated from where R , defined as the reflection from the surface, is a measure of the isotropic response equal to I S + I P . In our experiment, the probe beam is linearly polarized along the direction that produces maximum polarization activity. This is determined by the controlled experiment of probe polarization dependence, which rotates the polarization plane along one of the tetragonal crystal vectors. The probe focus diameter is ~200 μm, which is smaller than the length of elongated strips from twinned domains [5] . This allows to optically probe the index anisotropy even in unstrained crystals using highly sensitive laser-based polarimetry, as clearly demonstrated in Fig. 1c . Ultrafast polarimetry measurements For time-resolved measurements, a Ti:Sapphire amplifier with centre wavelength of 800 nm (1.55 eV), pulse duration of ~80 fs at the sample position and 1 kHz repetition rate was separated into pump and probe beams. The probe was frequency—doubled to 400 nm (3.1 eV) with a pulse duration of ~120 fs. This photon energy measures the nematic-order parameter φ , as demonstrated by the static measurement shown in Fig. 1c . This two—color pump—probe geometry was used to minimize the contamination of polarization signals during ultrafast time scales, for example, by dichroic bleaching, spectral weight transfer associated with pump-induced Fermi-surface reconstruction and transient filling of the mid-infrared SDW gaps and so on (for example, Stojchevska et al. [21] showed that near-infrared transient polarization signals persist far above all transition temperatures independent of doping). Lattice and electron relaxation dynamics are measured by the pump-induced optical reflectivity change Δ R / R . Small polarization or optical reflection changes were sampled as function of pump and probe delay by synchronously chopping the pump beam at 500 Hz and detecting the intensity change between consecutive pulses. Justification of the magnetic–nematic origin of transient polarization signals First, in our case, the relative variation of the anisotropic change is more than 100 times larger than that of the isotropic response. This huge magnitude difference makes a very strong case that the ellipticity change probes the genuine in-plane symmetry breaking of the magnetic–nematic phase. Second, the magnetic–nematic origin of the fs anisotropic response is further confirmed by controlled measurements showing a complete overlap of the pump-induced rotation ΔΘ( t ) and ellipticity Δ η ( t ) changes ( Supplementary Fig. 4 ). Any other non-magnetic contribution would cause discrepancy between the temporal profiles of the rotation angle and ellipticity, and vice versa. Further study is needed to investigate and understand the microscopic origins of the transient ellipticity signals and its distinct difference from isotropic signals, for example, a thorough comparison with time-/angle-resolved photoemission spectroscopy to study dynamics of orbital polarization and time-resolved X-ray scattering to follow dynamics of SDW orders. Theoretical modelling of the nematic-order parameter φ Here the nematic-order parameter φ is the scalar product of the two sublattice Neel vectors that make up the long-range order below T N : φ = < M 1 · M 2 > . The important aspect of this Ising-spin nematic phase is that long-range order of φ occurs already above the Neel temperature, that is, in a regime where the magnetic-order parameters still vanish < M 1 >=< M 2 >=0 (ref. 4 ). We follow the model extensively discussed by Fernandes et al. [4] to obtain the static nematic-order parameter φ as function of temperature (red line, Fig. 2b ). In this approach, the existence of a doubly degenerate magnetic ground state—stripes with either ( π , 0) or (0, π ) modulation—combined with strong-enough magnetic fluctuations gives rise to an Ising-nematic state, which spontaneously breaks the tetragonal symmetry of the system already in the paramagnetic state ( Supplementary Note 2 ). Theoretical modelling of ultrafast dynamics We model the obtained ultrafast dynamics with a 3T model. The set of coupled differential equations for energy flow are of the form below for three reservoirs with corresponding specific heat coefficients C e,m,l and coupling constants g ij (= g ji ): P ( t ) represents the pumping rate by the 80 fs Gaussian laser pulses over the excited volume. The pump fluence is 172 μJ cm −2 and absorbed fluence 67 μJ cm −2 after taking into account surface and cryostat window reflection loss. This corresponds to energy density of 673 J mol −1 deposited by the 80 fs Gaussian laser pulses over the excited volume into the sample. This is used as the input value for P ( t ) in the 3T model. The electronic specific heat is given by C e = γ e T e + C sc , where γ e =6.1 × 10 2 mJ m −3 ˙K 2 and C sc =2.475 × 10 2 mJ m −3 ˙K is the albeit small, average superconducting contribution acting only below T C . The lattice specific heat, C l , was determined from the Debye model with β =10 J m −3 ˙K 4 , whereas the magnetic–nematic specific heat C m was calculated from C m = C total − C e − C l . For the 3T model, we numerically solved the system of equations simultaneously via fourth- and fifth-order Runge–Kutta formulae to make error estimates and adjust the time step accordingly, and extracted the best-fit coupling constants to be: g em =3.16 × 10 17 W m −3 ˙K, g ml =13.3 × 10 17 W m −3 ˙K and g el =0.033 × 10 17 W m −3 ˙K. Error bars for g em , g ml and g el are 0.58 × 10 17 , 1.66 × 10 17 and 0.13 × 10 17 W m −3 ˙K, respectively. The inset shows the same simulation for nickel using the well-established parameters in the literature [24] . The coupling constants for nickel are g el =8 × 10 17 W m −3 ˙K, g em =6 × 10 17 W m −3 ˙K, g lm =0.3 × 10 17 W m −3 ˙K. How to cite this article: Patz, A. et al. Ultrafast observation of critical nematic fluctuations and giant magnetoelastic coupling in iron pnictides. Nat. Commun. 5:3229 doi: 10.1038/ncomms4229 (2014).